Acyl radical to rhodacycle addition and cyclization relay to access butterfly flavylium fluorophores Transition metal-catalyzed C–H activation and radical reactions are two versatile strategies to construct diverse organic skeletons. Here we show the construction of a class of flavylium fluorophores via the merge of radical chemistry and C–H activation starting from (hetero)aryl ketones and alkynes. This protocol is not only applicable to aryl ketones but also to heteroaryl ketones such as thiophene, benzothiophene and benzofuran, thus leading to structural diversity. Mechanism studies, including control experiments, intermediate separation, radical trapping, EPR and ESI-HRMS experiments, demonstrate that the key step lies in the addition of the acyl radical generated by the copper-catalyzed C–C bond cleavage of aryl ketone to the rhodacycle formed via the C–H activation of aryl ketone. The flavylium fluorophores feature butterfly symmetrical configuration, nearly planar skeleton and delocalized positive charge, and exhibit intriguing photophysical properties, such as tunable absorption and emission wavelengths and high quantum yields. Due to attractive electronic, optical, electrochemical and magnetic properties, organic fluorophores have been considered as promising candidates for applications, such as fluorescent markers, photosensitizers, nonlinear optical materials and nano-electronic devices [1] , [2] , [3] , [4] , [5] , [6] , [7] , [8] , [9] , [10] , [11] , [12] , [13] . Therefore, diverse kinds of organic fluorophores have been discovered and developed, among which nitrogen-based porphyrins [1] , [2] , BODIPYs [3] , [4] , [5] and cyanine derivatives [6] , [7] exhibit extensive and outstanding properties (Fig. 1a ). In recent years, oxygen-doped fluorophores based on pyrylium framework begin to attract attention because of tunable emission wavelength, high quantum yield and water solubility, making them as ideal optical-imaging reagents (Fig. 1b ) [8] , [9] , [10] , [11] , [12] , [13] . From both the fundamental and application viewpoints, a study of the structural diversity of organic fluorophores is doubtlessly of great importance. Fig. 1: Representative organic fluorophores. a Nitrogen-based fluorophores. b Oxygen-based fluorophores. Full size image Transition metal-catalyzed C–H activation and radical reactions have been developed as two versatile tools for the construction of organic functional skeletons [14] , [15] , [16] , [17] , [18] , [19] , [20] , [21] , [22] , [23] , [24] , [25] , [26] , [27] , [28] , [29] , [30] , [31] , [32] , [33] , [34] , [35] . The metal-catalyzed C–H activation reactions proceed via the formation of carbon–metal bond, typically classified as charged species—involving ionic reactions, while the key step of the radical reactions involves an electrophilic addition of a radical species to arene, alkene, or alkyne. Undoubtedly, the combination of ionic and radical reactions would create new chemical transformations and thereby produce complex molecules with high reaction efficiency. Despite an appealing strategy, it is challenging to achieve a well-organized reaction relay because the presence of the highly reactive radical species may give rise to an uncontrollable, complicated reaction process. Given the weak coordinating ability and keto–enol tautomerism, as well as easily being oxidized to radical species, aryl ketones are considered as an ideal element to implement diverse chemical transformations [20] , [21] , [22] , [23] , [32] , [33] . By using aryl ketones and alkynes as substrates, Glorius and Cheng independently reported the rhodium-catalyzed C2–H activation/annulation reactions to deliver indenol and fulvene derivatives [20] , [21] . In our previous work, carbohelicenes were synthesized by a C–H activation/radical approach/C–H activation relay of α-acetylnaphthalenes with alkynes [35] . Herein, we describe the addition of an acyl radical generated by the copper-catalyzed sequential oxidation/C–C bond cleavage of (hetero)arylketones to the rhodacycle to produce butterfly flavylium fluorophores (BFFs) with symmetrical and nearly planar skeleton with delocalized positive charge (Fig. 2 ). Fig. 2: Merging radical chemistry with C–H activation to construct BFFs. a In this report, one step synthesis of BFFs. b The proposed reaction pathway. Full size image 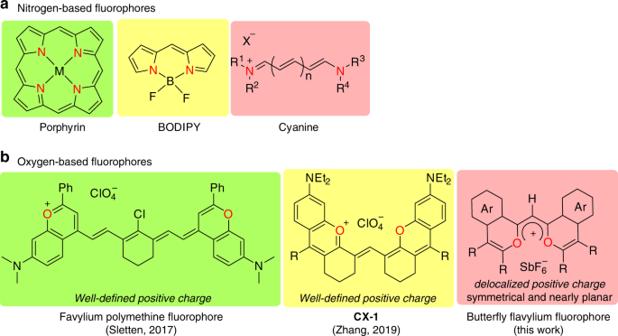Fig. 1: Representative organic fluorophores. aNitrogen-based fluorophores.bOxygen-based fluorophores. Analysis of structure and DFT calculation In the investigation of the reaction of 4-methoxyacetophenone with diphenylacetylene, the BFF 3aa was unexpectedly isolated in 8% yield by using 5 mol% of [Cp*RhCl 2 ] 2 as the catalyst, Ag 2 O as the oxidant, Cu(OAc) 2 ·H 2 O as the additive, and DCE as the solvent in the presence of 20 mol% of AgSbF 6 at 150 °C (Supplementary Table 1 , entry 1). X-ray single crystal analysis of 3aa shows a nearly planar skeleton with a little angle of 11.6° between the two pyrylium rings (Fig. 3a, b ). The length of C2–C3 bond (1.389(5) Å) is close to that of C3–C4 bond (1.372(5) Å), which are between the lengths of C–C single bond (1.455 Å) and C = C double bond (1.326 Å) [36] . The 1 H NMR spectrum of 3aa shows a symmetrical configuration, suggesting that the positive charge is delocalized equally around the skeleton. In addition, density functional theory (DFT) calculation was employed to evaluate the intrinsic characteristic of cationic 3aa (Supplementary Data 1 ) [37] , [38] . As shown in Fig. 3c, d , the natural population analysis and natural bond orbital (NBO) atomic charge distribution further illustrate that the positive charge of 3aa is mostly delocalized by the two pyrylium rings. Fig. 3: X-ray single crystal diffraction analysis and DFT calculation of 3aa. a Top view of X-ray single crystal structure of 3aa . b Side view of X-ray single crystal structure of 3aa . c Electrostatic potential maps of 3aa . d Calculated NBO atomic charge distribution of cationic 3aa . Full size image Optimization of the reaction conditions With the butterfly flavylium scaffold in hand, optimization of the reaction conditions was next conducted (Supplementary Table 1 ). Considering the zwitterionic form of the product, 1.5 equivalents of NaSbF 6 were added into the reaction system, improving the yield of 3aa to 45% (Supplementary Table 1 , entry 3). The copper salt is important for this reaction and no desired product could be detected without the addition of copper salt (Supplementary Table 1 , entry 4). Subsequently, various copper species, such as CuBr 2 , CuO, CuCl, Cu(OAc), and Cu 2 O were screened (Supplementary Table 1 , entries 5–9). 3aa was obtained in 49% yield when 0.04 mmol of Cu(OAc) 2 ·H 2 O was used (Supplementary Table 1 , entry 10). Oxidant Ag 2 CO 3 could further improve the yield of 3aa to 63% (Supplementary Table 1 , entry 15). Solvents are critical for this reaction and other solvents, such as toluene, tetrahydrofuran, 1, 4-dioxane, and N , N -dimethylformamide did not deliver the product (Supplementary Table 1 , entries 17–20). The yield of 3aa could reach 73% by decreasing the temperature from 150 to 100 °C (Supplementary Table 1 , entry 24). Substrate scope To assemble a structurally diverse library of the BFFs, the substrate scope was conducted. As shown in Fig. 4 , the cascade annulation of (hetero)aryl ketones with alkynes allowed a relatively broad substrate scope, producing a diverse family of BFFs in moderate to good yields. The aryl ketones with an electron-donating group at the para position such as N,N -dimethyl could deliver the desired fluorophore ( 3ba ) in 39% yield. 3-Methylacetophenone and 3,4-dimethoxyacetophenone could give the corresponding fluorophores, but the pure products were not obtained because of their instability during column chromatography. Delightedly, the heteroaryl ketones such as 2-acetylthiophene, 2-acetylbenzo[ b ]thiophene, 2-acetylbenzo[ b ]furan, and 3-acetylbenzo[ b ]thiophene could afford the corresponding fluorophores ( 3da - 3ga ) in moderate yields. The good compatibility of heteroaryl ketones enriches the structural diversity. Next, the scope of the alkyne derivatives was investigated. The electron-donating group such as methyl and methoxy could be tolerated, producing the desired products ( 3ab - 3ac ) in moderate to good yields. The unsymmetrical alkyl aryl alkyne delivered 3ad with a good regioselectivity and other isomers were not detected. Fig. 4: Substrate scope. Reaction conditions: 1 (0.2 mmol), 2 (0.3 mmol), [Cp*RhCl 2 ] 2 (5 mol%), AgSbF 6 (20 mol%), Ag 2 CO 3 (0.3 mmol), Cu(OAc) 2 ·H 2 O (0.04 mmol), NaSbF 6 (0.15 mmol), and DCE (0.5 mL) at 100 °C for 12 h under N 2. † At 75 °C for 4 h. ‡ At 150 °C. Full size image Mechanism of investigation To get a clearer perception of this cascade process, a set of control experiments were performed (Fig. 5 ). Firstly, under the standard reaction conditions, acetophenone, respectively, delivered the BFF 3ca in 22% yield at 100 °C and 40% yield at 150 °C, while 1,3-diphenylpropane-1,3-dione did not deliver the corresponding product either at 100 or 150 °C (Fig. 5a, b ). These results indicated that 1,3-dicarbonyl compound was not the intermediate of this reaction. Secondly, under otherwise identical reaction conditions, the absence of counteranion source NaSbF 6 led to 3aa in 12% yield and the fulvene derivative 4aa in 28% yield (Fig. 5c ). Under the standard reaction conditions, the reaction of 1a with 2a could deliver a trace amount of the fulvene derivative 4aa . The formation of 4aa demonstrated that the C2–H activation process of arylketone existed in this reaction system. The ESI-HRMS experiment did not detect 5aa , implying that the cascade reaction might be a successive process rather than a step by step process (Fig. 5c ). In a step by step process, a stable reaction intermediate could be isolated through condition control and the final product could be obtained in an acceptable yield by using the reaction intermediate as the starting material. Thirdly, under the standard reaction conditions, the reaction of 1a , 2a , and 4-methoxybenzoyl formic acid gave a mixture of 3ca and the unsymmetric product 6ca , which was detected by ESI-HRMS (Fig. 5d and Supplementary Fig. 3 ). This result suggested that the benzoylformic acid could be one of the reaction intermediates and the deprivation of the carbon atom could be related to the decarboxylation process. Fig. 5: Control experiments for the reaction mechanism. a The reaction of 1,3-diphenylpropane-1,3-dione with 2a was performed under standard reaction conditions. b The reaction of 1c with 2a was performed under the standard reaction conditions at 100 or 150 °C. c The reaction of 1a with 2a was performed without the addition of the extra anion source NaSbF 6 . d The reaction of 1c , 2a , and 4-methoxybenzoyl formic acid was performed under the standard reaction conditions. Full size image Based on the above results, we infer that this transformation might involve two main processes: (a) the generation of rhodacycle by the C2–H activation of arylketone; and (b) the generation of acyl radical by the oxidation/decarboxylation sequence of arylketone. To gain more insights into the radical process, radical trapping experiments were carried out. The yield of 3aa decreased from 52% to trace with increasing amount of radical quencher (2,2,6,6-tetramethylpiperidin-1-yl)oxyl (TEMPO), suggesting the possible radical pathway (Fig. 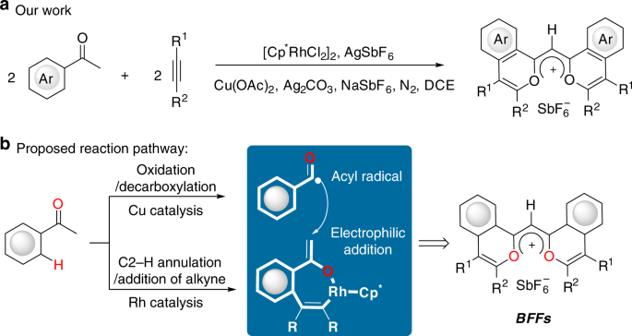Fig. 2: Merging radical chemistry with C–H activation to construct BFFs. aIn this report, one step synthesis of BFFs.bThe proposed reaction pathway. 6a and Supplementary Table 2 ). Subsequently, EPR analysis indicated that the reaction of 1a with 2a was EPR-active, while no signals were observed in the absence of both 1a and 2a (Fig. 6b, c and Supplementary Fig. 6a, b ). Under the standard reaction conditions, the product 3aa had only a weak EPR signal (Supplementary Fig. 6c ). Furthermore, the reaction of 1e , 2a and TEMPO could deliver the isocoumarin product 7ea in 39% yield, while only a trace amount of 7ea could be detected without the addition of TEMPO (Fig. 6d ). This result indicated that the adduct of acyl radical with TEMPO could be the reaction intermediate for the generation of 7ea (for details, see Supplementary Fig. 4 ). In addition, without the addition of catalyst [Cp*RhCl 2 ] 2 , the reaction of 1e , 2a and TEMPO could produce 8ea in 18% yield, demonstrating the generation of acyl radical (Fig. 6e and Supplementary Fig. 5 ). These results clearly demonstrated that the acyl radical species is involved in the cascade reaction. Fig. 6: Detection of radical intermediates. a Radical trapping experiments. b EPR experiments of the reaction 1a with 2a . c EPR spectrum of the reaction mixture of 1a and 2a under standard reaction conditions. d The reaction of 1e , 2a , and TEMPO under the standard reaction conditions. e The reaction of 1e , 2a , and TEMPO without the addition of catalyst [Cp*RhCl 2 ] 2 . Full size image Based on the experimental observations and the reported literature, the reaction pathway is proposed in Fig. 7 . Firstly, the reactive [Rh III Cp * ] A is formed via the reaction of [Cp*RhCl 2 ] 2 with AgSbF 6 , followed by the cyclometalation and alkyne insertion. The resulting intermediate C could undergo a keto–enol tautomerism to generate the intermediate D , which is more easily to be trapped by a radical species. At the same time, the (hetero)aryl ketone is oxidized to (hetero)aryl glyoxylic acid, followed by the generation of acyl radical through a decarboxylation under copper catalysis [39] , [40] . The selective electrophilic addition of the acyl radical to the rhodacycle D gives the radical species E , followed by the sequential oxidation and deprotonation process to form intermediate F . In the synthesis of indenol and fulvene derivatives reported by Glorius, the catalytic Cu(OAc) 2 ·H 2 O plays the role in the release of the rhodium catalyst in a transmetalation event [20] . We propose that one of the key roles of Cu(OAc) 2 ·H 2 O is to promote the intramolecular rhodium migration, accompanied by the oxidation of Rh(I) to Rh(III) and the C–H activation of another (hetero)arylketone to form intermediate G . The second alkyne inserts into G to produce H , followed by a reductive elimination to yield the butterfly flavylium fluorophore. By the oxidation of Ag 2 CO 3 , the active Rh (III) species is regenerated. There is another possible pathway from intermediate B to F as shown in Fig. 7 . The acyl radical may attack the intermediate J generated by a keto–enol tautomerism of B prior to the first alkyne insertion. Fig. 7: Plausible catalytic cycle. The possible mechanism involves the Rh-catalyzed C2–H activation of aryl ketone to generate the rhadocycle and the Cu-catalyzed oxidation/C–C bond cleavage of aryl ketone to produce the acyl radical. 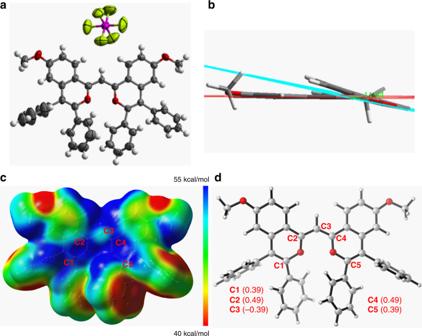Fig. 3: X-ray single crystal diffraction analysis and DFT calculation of 3aa. aTop view of X-ray single crystal structure of3aa.bSide view of X-ray single crystal structure of3aa.cElectrostatic potential maps of3aa.dCalculated NBO atomic charge distribution of cationic3aa. Full size image Photophysical properties of BFFs With the diverse BFFs in hand, the photophysical properties of fluorophores, including UV–Vis absorption, fluorescence emission, extinction coefficients, excitation, and quantum yield, were measured in CH 2 Cl 2 (Supplementary Table 3 and Supplementary Fig. 7 ). As shown in Fig. 8 and Supplementary Table 3 , the BFFs show tunable absorption and emission wavelengths and high quantum yields in CH 2 Cl 2 . The quantum yields of the fluorophores 3ca , 3ea , 3fa , and 3ac could reach 46%, 59%, 63%, and 49% even with emission maxima of 626, 656, 660, and 631 nm, respectively. Fig. 8: Absorption and emission spectra of the BFFs in CH 2 Cl 2 at 40.0 μM. a The absorption spectra of 3aa , 3ba , 3ca , 3da , and 3ea . b The absorption spectra of 3fa , 3ga , 3ab , 3ac and 3ad . c The emission spectra of all BFFs. Full size image In summary, a class of BFFs has been developed through the merging of C–H activation and radical chemistry. Because both (hetero)arylketones and alkynes are easily available and structurally diverse, the structures of the BFFs are easily subjected to chemical modification. 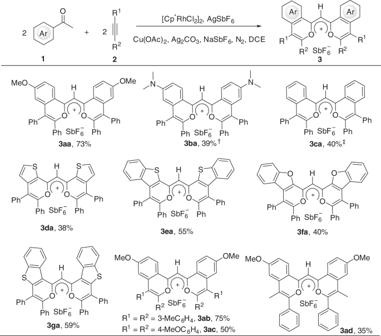Fig. 4: Substrate scope. Reaction conditions:1(0.2 mmol),2(0.3 mmol), [Cp*RhCl2]2(5 mol%), AgSbF6(20 mol%), Ag2CO3(0.3 mmol), Cu(OAc)2·H2O (0.04 mmol), NaSbF6(0.15 mmol), and DCE (0.5 mL) at 100 °C for 12 h under N2.†At 75 °C for 4 h.‡At 150 °C. These fluorophores exhibit intriguing photophysical properties, such as tunable absorption and emission wavelengths, high quantum yield and zwitterionic form, rendering them potential applications as luminescence materials. The rapid gateway to BFFs described herein has further exemplified the power of the combination of C–H activation and radical chemistry in the exploration of organic functional materials. General procedure for the synthesis of BFFs A Schlenk tube with a magnetic stir bar was charged with [Cp*RhCl 2 ] 2 (0.005 mmol), AgSbF 6 (0.02 mmol), Ag 2 CO 3 (0.3 mmol), Cu(OAc) 2 ·H 2 O (0.04 mmol), NaSbF 6 (0.15 mmol), arylketone (0.2 mmol), alkyne (0.3 mmol), and DCE (0.5 mL) under an N 2 atmosphere. 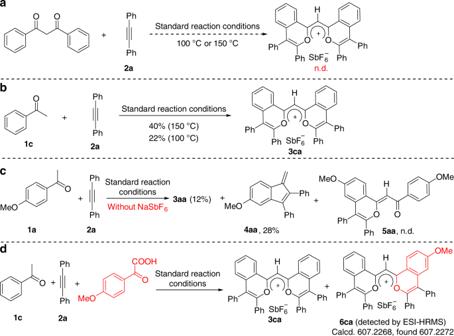Fig. 5: Control experiments for the reaction mechanism. aThe reaction of 1,3-diphenylpropane-1,3-dione with2awas performed under standard reaction conditions.bThe reaction of1cwith2awas performed under the standard reaction conditions at 100 or 150 °C.cThe reaction of1awith2awas performed without the addition of the extra anion source NaSbF6.dThe reaction of1c,2a, and 4-methoxybenzoyl formic acid was performed under the standard reaction conditions. The resulting solution was stirred at room temperature for 10 min and then at the indicated temperature for the indicated time. 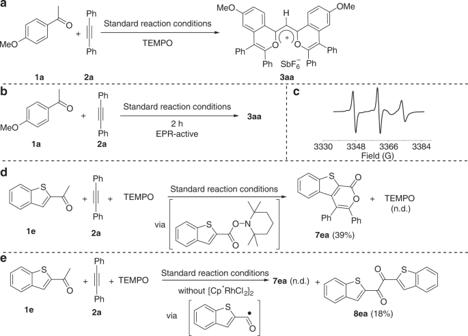Fig. 6: Detection of radical intermediates. aRadical trapping experiments.bEPR experiments of the reaction1awith2a.cEPR spectrum of the reaction mixture of1aand2aunder standard reaction conditions.dThe reaction of1e,2a, and TEMPO under the standard reaction conditions.eThe reaction of1e,2a, and TEMPO without the addition of catalyst [Cp*RhCl2]2. The resulting solution was cooled to ambient temperature, diluted with 10 mL of dichloromethane. The obtained organic extracts was evaporated under reduced pressure and the residue was absorbed into small amounts of silica gel. Purification was performed by column chromatography on silica gel to provide product 3 . 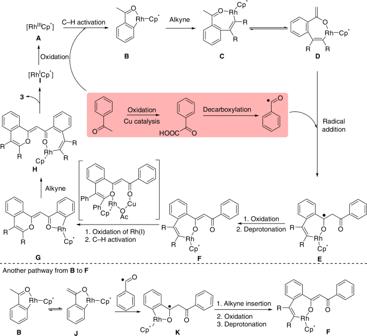Fig. 7: Plausible catalytic cycle. The possible mechanism involves the Rh-catalyzed C2–H activation of aryl ketone to generate the rhadocycle and the Cu-catalyzed oxidation/C–C bond cleavage of aryl ketone to produce the acyl radical. 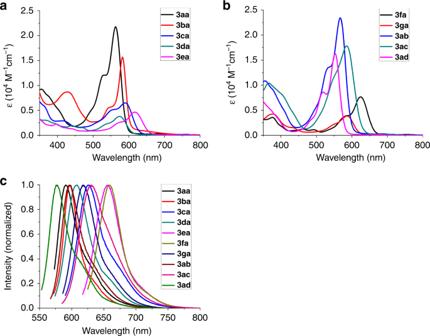Fig. 8: Absorption and emission spectra of the BFFs in CH2Cl2at 40.0 μM. aThe absorption spectra of3aa,3ba,3ca,3da, and3ea.bThe absorption spectra of3fa,3ga,3ab,3acand3ad.cThe emission spectra of all BFFs. The reaction vessel is under pressure and could possibly explode because of higher reaction temperature than the boiling point of DCE.